Phosphorylation of EXO1 by CDKs 1 and 2 regulates DNA end resection and repair pathway choice Resection of DNA double-strand breaks (DSBs) is a pivotal step during which the choice between NHEJ and HR DNA repair pathways is made. Although CDKs are known to control initiation of resection, their role in regulating long-range resection remains elusive. Here we show that CDKs 1/2 phosphorylate the long-range resection nuclease EXO1 at four C-terminal S/TP sites during S/G2 phases of the cell cycle. Impairment of EXO1 phosphorylation attenuates resection, chromosomal integrity, cell survival and HR, but augments NHEJ upon DNA damage. In contrast, cells expressing phospho-mimic EXO1 are proficient in resection even after CDK inhibition and favour HR over NHEJ. Mutation of cyclin-binding sites on EXO1 attenuates CDK binding and EXO1 phosphorylation, causing a resection defect that can be rescued by phospho-mimic mutations. Mechanistically, phosphorylation of EXO1 augments its recruitment to DNA breaks possibly via interactions with BRCA1. In summary, phosphorylation of EXO1 by CDKs is a novel mechanism regulating repair pathway choice. The integrity of our genome is constantly threatened by DNA double-strand breaks (DSBs). Two major pathways have evolved to repair these breaks [1] . Non-homologous end joining (NHEJ) is an error-prone pathway during which DNA ends are ligated independently of a template, whereas homologous recombination (HR) is an error-free pathway that uses the intact sister chromatid as a template for repair. Cell cycle regulation of these two pathways is critical for the maintenance of genomic integrity. Suppression of HR in G1 prevents loss of heterozygosity and chromosomal rearrangements arising from recombination with the homologous chromosome or non-allelic homologous loci, respectively. On the other hand, promotion of HR in S and G2 phases ensures accurate repair, especially that of one-ended replication fork-associated breaks. However, the underlying mechanisms of cell cycle regulation of NHEJ and HR pathways are not completely worked out. Coupling DNA repair machineries to the engine that drives the cell cycle, namely, cyclin-dependent kinases (CDKs) in complex with their cyclin partners [2] , is an efficient way to achieve cell cycle regulation of DSB repair. It is becoming increasingly clear that the CDKs that promote cell cycle progression through S and G2 phases concomitantly promote HR in these phases by activating the first step in recombination, viz. DNA end resection [3] , [4] . DNA end resection in the 5′–3′ direction results in the formation of a 3′-OH single-stranded tail that is first coated with replication protein A (RPA), which is then exchanged for Rad51 to form a recombinogenic nucleofilament. Resection is a key step at which ‘repair pathway choice’, the choice between NHEJ and HR, can be enforced by the cell as the generation of single-stranded DNA (ssDNA) would favour HR and concomitantly disfavour NHEJ by stymieing the binding of NHEJ proteins. A ‘two-step’ model of resection has been formulated, based mainly on studies in yeast [3] , [5] . The first step, ‘initiation of resection’, involves the removal of ~50–100 bases of DNA from the 5′-end by the MRX/MRN complex (Mre11–Rad50–Xrs2 in yeast and Mre11–Rad50–Nbs1 in humans) in conjunction with Sae2/CtBP-interacting protein (CtIP) [6] , [7] , [8] , [9] . The second step, ‘long-range resection’, is carried out by two alternate pathways involving the 5′–3′ exonuclease Exo1 on one hand, and the helicase–topoisomerase complex Sgs1–Top3–Rmi1/BLM–TOPIIIα–RMI1-2 in concert with the nuclease Dna2 on the other hand. The current understanding is that CDKs control DNA end resection and repair pathway choice by promoting the initiation of resection via phosphorylation of Sae2/CtIP and Nbs1 (refs 10 , 11 , 12 , 13 , 14 , 15 , 16 ). Here we describe a novel mechanism by which CDKs control repair pathway choice in human cells that involves regulation of long-range resection via phosphorylation of EXO1. EXO1 is phosphorylated by CDKs 1 and 2 in S and G2 phases We have previously shown that EXO1 plays a major role in resection and HR in human cells [17] , [18] , [19] , [20] , making it a plausible candidate for regulation by CDKs in a cell cycle-dependent manner. To examine this possibility, HEK-293 cells ectopically expressing V5-tagged EXO1 were synchronized in different phases of the cell cycle ( Supplementary Fig. 1a ). EXO1 was immunoprecipitated (IP) with anti-V5 antibody and western blotted with anti-phospho-(Ser) or anti-phospho-(Thr) CDK substrate antibodies. We observed that EXO1 was increasingly phosphorylated as cells traversed the cell cycle from G1, through S, to G2 ( Fig. 1a ). No increase in EXO1 phosphorylation was seen on treating cells with ionizing radiation (IR) or ultraviolet indicating that the increase in EXO1 phosphorylation seen with cell cycle progression was not due to any genotoxic stress caused by cell synchronization methods ( Supplementary Fig. 1b ). 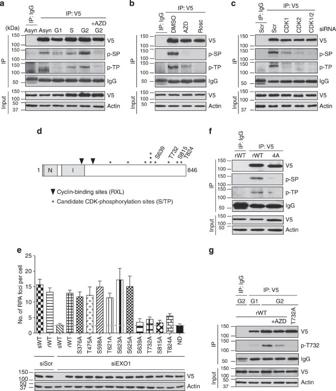Figure 1: EXO1 is phosphorylated by CDKs 1 and 2 in S and G2 phases. (a) HEK-293 cells expressing V5-EXO1 were synchronized in different phases of the cell cycle. EXO1 was immunoprecipitated (IP) with anti-V5 antibody and western blotted with anti-phospho-Ser (p-SP) or anti-phospho-Thr (p-TP) CDK substrate antibodies, as indicated. ‘+AZD’ indicates cells pre-treated with the CDK inhibitor AZD5438 before analysis. (b) HEK-293 cells expressing V5-EXO1, synchronized in G2, were pre-treated with CDK inhibitors, AZD5438 or roscovitine, before analysis of EXO1 phosphorylation by IP-western. (c) HEK-293 cells expressing V5-EXO1, with siRNA-mediated depletion of CDK1 and/or CDK2, were synchronized in G2 and EXO1 phosphorylation status determined by IP-western. Scr denotes scrambled siRNA used as a control. (d) Schematic of human EXO1 with asterisks indicating location of S/TP sites. Sites determined in this study to be important for resection are numbered. Locations of cyclin-binding (Cy) sites are indicated by solid triangles. N-terminal (N) and internal (I) catalytic domains are indicated. (e) U2OS cells were depleted of endogenous EXO1 using siRNA and complemented with siRNA-resistant wild-type EXO1 (rWT) or EXO1 individually mutated at S/TP sites, as indicated. Cells were screened for resection defects by quantifying IR-induced RPA foci. Average numbers of RPA foci per cell are plotted after subtracting background (average numbers of foci in mock-irradiated cells). Cells expressing siRNA-sensitive EXO1 (sWT) or siRNA-resistant nuclease dead EXO1 (ND) served as resection-defective controls (dashed line demarcates basal levels of RPA foci in these cells). Western blot shows comparable expression of EXO1 mutants and depletion of sWT-EXO1 by siRNA. (f) HEK-293 cells expressing WT-EXO1 or EXO1 with all four C-terminal S/TP sites mutated to Ala (4A-EXO1) were synchronized in G2, and EXO1 phosphorylation status determined by IP-western. (g) HEK-293 cells expressing WT-EXO1 or EXO1 with a T732A point mutation were synchronized in G1 or G2, as indicated, and EXO1 phosphorylation at the T732 site was determined by IP-western with anti-phospho-EXO1 (p-T732) antibody. All experiments were replicated three times. Error bars depict s.e.m. See alsoSupplementary Fig. 1. Phosphorylation of EXO1 in cells synchronized in G2 was attenuated by the CDK inhibitors AZD5438 and roscovitine [21] , [22] , both of which inhibit CDKs 1 and 2, the principal CDKs driving progression through S and G2 phases [2] ( Fig 1a,b ; Supplementary Fig. 1c ). Phosphorylation of EXO1 in cells synchronized in G2 was also attenuated on short interfering RNA (siRNA)-mediated depletion of CDKs 1 and 2 ( Fig. 1c ; Supplementary Fig. 1d ). Depletion of CDK 1 and/or 2 did not significantly alter cell cycle profiles ( Supplementary Fig. 1e ); hence, the observed reduction in EXO1 phosphorylation was not due to a reduction in the total population in S and G2. These observations indicated that EXO1 is hyperphosphorylated by CDKs 1 and 2 in S and G2 phases of the cell cycle and hinted that EXO1 may be regulated by CDKs. Figure 1: EXO1 is phosphorylated by CDKs 1 and 2 in S and G2 phases. ( a ) HEK-293 cells expressing V5-EXO1 were synchronized in different phases of the cell cycle. EXO1 was immunoprecipitated (IP) with anti-V5 antibody and western blotted with anti-phospho-Ser (p-SP) or anti-phospho-Thr (p-TP) CDK substrate antibodies, as indicated. ‘+AZD’ indicates cells pre-treated with the CDK inhibitor AZD5438 before analysis. ( b ) HEK-293 cells expressing V5-EXO1, synchronized in G2, were pre-treated with CDK inhibitors, AZD5438 or roscovitine, before analysis of EXO1 phosphorylation by IP-western. ( c ) HEK-293 cells expressing V5-EXO1, with siRNA-mediated depletion of CDK1 and/or CDK2, were synchronized in G2 and EXO1 phosphorylation status determined by IP-western. Scr denotes scrambled siRNA used as a control. ( d ) Schematic of human EXO1 with asterisks indicating location of S/TP sites. Sites determined in this study to be important for resection are numbered. Locations of cyclin-binding (Cy) sites are indicated by solid triangles. N-terminal (N) and internal (I) catalytic domains are indicated. ( e ) U2OS cells were depleted of endogenous EXO1 using siRNA and complemented with siRNA-resistant wild-type EXO1 (rWT) or EXO1 individually mutated at S/TP sites, as indicated. Cells were screened for resection defects by quantifying IR-induced RPA foci. Average numbers of RPA foci per cell are plotted after subtracting background (average numbers of foci in mock-irradiated cells). Cells expressing siRNA-sensitive EXO1 (sWT) or siRNA-resistant nuclease dead EXO1 (ND) served as resection-defective controls (dashed line demarcates basal levels of RPA foci in these cells). Western blot shows comparable expression of EXO1 mutants and depletion of sWT-EXO1 by siRNA. ( f ) HEK-293 cells expressing WT-EXO1 or EXO1 with all four C-terminal S/TP sites mutated to Ala (4A-EXO1) were synchronized in G2, and EXO1 phosphorylation status determined by IP-western. ( g ) HEK-293 cells expressing WT-EXO1 or EXO1 with a T732A point mutation were synchronized in G1 or G2, as indicated, and EXO1 phosphorylation at the T732 site was determined by IP-western with anti-phospho-EXO1 (p-T732) antibody. All experiments were replicated three times. Error bars depict s.e.m. See also Supplementary Fig. 1 . Full size image Human EXO1 bears 10 putative S/TP CDK phosphorylation sites, 2 of which (T732 and S815) conform to the optimal CDK-recognition motif, (S/T)PX(K/R) [23] ( Fig. 1d ). To identify S/TP sites that might be important for resection, U2OS cells with siRNA-mediated depletion of endogenous EXO1 were complemented with 10 different siRNA-resistant EXO1 constructs that were individually mutated to non-phosphorylatable Ala at each of these putative phosphorylation sites. siRNA-resistant wild-type EXO1 (rWT-EXO1) served as a positive control, while siRNA-sensitive wild-type EXO1 (sWT-EXO1) and nuclease dead EXO1 bearing a D173A mutation [24] (ND-EXO1) served as negative controls. Cells were screened for resection defects by quantifying RPA foci after irradiation, as described previously [19] (see legends to Supplementary Fig. 1f–h for description of the screen and controls). We found that individual mutations of the four carboxy-terminal S/TP sites (S639, T732, S815 and T824) resulted in resection defects as evidenced by reduced numbers of RPA foci ( Fig. 1e ). Mutation of all four sites to Ala (4A-EXO1) eliminated EXO1 detection by anti-CDK substrate antibodies ( Fig. 1f ). However, negligible reduction was observed with individual mutations of these four sites probably because the anti-CDK substrate antibodies are not site specific and would recognize multiple phosphorylated S/TP sites on the same protein ( Supplementary Fig. 1i ). Therefore, to directly demonstrate phosphorylation of specific S/TP sites in vivo , we attempted to generate phospho-specific antibodies against these sites, and were successful in raising antibodies to phospho-T732 ( Supplementary Fig. 1j,k ). In IP-westerns, the anti-p-T732 antibody could recognize WT-EXO1 but not the non-phosphorylatable T732A mutant, confirming the specificity of this antibody ( Fig. 1g ). Phosphorylation of EXO1 at T732 was cell cycle- and CDK-dependent, with a higher level of phosphorylation observed in G2 that was attenuated on pretreatment of cells with the CDK inhibitor AZD5438 ( Fig. 1g ). Akin to V5-tagged EXO1, endogenous EXO1 in these cells was also phosphorylated in a cell cycle- and CDK-dependent manner ( Supplementary Fig. 1l ). Our results directly demonstrate that T732 of EXO1 is phosphorylated in vivo in a cell cycle- and CDK-dependent manner. Moreover, western blotting results with 4A-EXO1 ( Fig. 1f ) tentatively indicate that the other three identified sites are also phosphorylated in S/G2 phases, a supposition borne out by independent mass spectrometric analyses identifying S639 and S815 of EXO1 as bona fide phosphorylation targets in vivo [25] , [26] , [27] . Phosphorylation of EXO1 by CDKs promotes DNA end resection To definitively establish the role of these four sites in regulation of DSB resection and HR, we used three complementary assays involving quantification of RPA, 5-bromo-2′-deoxyuridine (BrdU)/ssDNA and Rad51 foci, and compared foci formation in cells expressing WT-EXO1, non-phosphorylatable 4A-EXO1 or phospho-mimic 4D-EXO1 (all four sites replaced with Asp). Cells expressing 4A-EXO1 were severely impaired in RPA foci formation after irradiation, similar to that seen in cells expressing ND-EXO1 ( Fig. 2a ; Supplementary Fig. 2a ), and this defect was more severe than that seen with EXO1 individually mutated at these four sites ( Fig. 1e ). Interestingly, cells expressing 4D-EXO1 were proficient in RPA foci formation and actually exhibited higher numbers of foci than cells expressing wild-type EXO1 (rWT-EXO1). The impairment in RPA foci formation on expression of 4A-EXO1 was clearly due to impaired DNA resection, directly quantified as IR-induced BrdU/ssDNA foci, as described previously [20] ( Fig. 2b ). The resection defect in cells expressing 4A-EXO1 resulted in a decrease in IR-induced Rad51 foci [17] in S/G2 cells (cyclin A positive [28] ), suggesting attenuated HR ( Fig. 2c ). The observed impairments in resection and HR were not due to perturbations of the cell cycle as assessed by flow cytometry ( Supplementary Fig. 2b ) or attenuation of the nuclease activity of 4A-EXO1 as assessed by in vitro nuclease assay ( Supplementary Fig. 2c ). 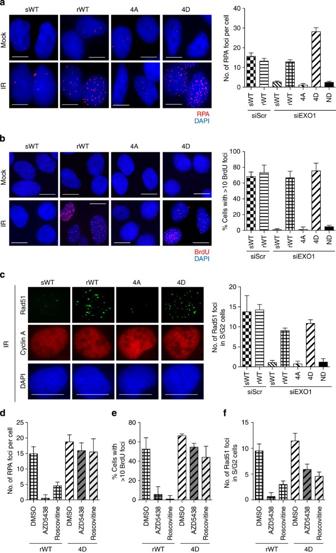Figure 2: Phosphorylation of EXO1 by CDKs promotes DNA end resection. (a) U2OS cells were depleted of endogenous EXO1 using siRNA and complemented with siRNA-sensitive wild-type EXO1 (sWT) or siRNA-resistant wild-type EXO1 (rWT), non-phosphorylatable mutant EXO1 (4A) or phospho-mimic EXO1 with all four C-terminal S/TP sites replaced with Asp (4D), as indicated. Representative images of mock-irradiated or irradiated (IR) cells immunostained with anti-RPA antibody (red) are shown. Nuclei were stained with 4',6-diamidino-2-phenylindole (blue). Plot shows average numbers of RPA foci per cell after subtracting background (average numbers of foci in mock-irradiated cells). (b) Representative images of mock-irradiated or irradiated cells immunostained for BrdU/ssDNA foci (red) are shown. Plot shows percentages of cells with more than 10 BrdU foci per nucleus after background subtraction. (c) Representative images of irradiated cells co-immunofluorescence stained with anti-cyclin A antibody (red) and anti-Rad51 antibody (green) are shown. Average numbers of Rad51 foci for cyclin A-positive (S/G2) nuclei are plotted after background subtraction. (d–f) Cells expressing rWT or 4D-EXO1 were pre-treated with CDK inhibitors (AZD5438 or roscovitine) or with DMSO as control, irradiated and assayed for RPA, BrdU or Rad51 foci, as indicated. Scale bar, 10 μm (for all images). All experiments were replicated three times. Error bars depict s.e.m. See alsoSupplementary Fig. 2. Figure 2: Phosphorylation of EXO1 by CDKs promotes DNA end resection. ( a ) U2OS cells were depleted of endogenous EXO1 using siRNA and complemented with siRNA-sensitive wild-type EXO1 (sWT) or siRNA-resistant wild-type EXO1 (rWT), non-phosphorylatable mutant EXO1 (4A) or phospho-mimic EXO1 with all four C-terminal S/TP sites replaced with Asp (4D), as indicated. Representative images of mock-irradiated or irradiated (IR) cells immunostained with anti-RPA antibody (red) are shown. Nuclei were stained with 4',6-diamidino-2-phenylindole (blue). Plot shows average numbers of RPA foci per cell after subtracting background (average numbers of foci in mock-irradiated cells). ( b ) Representative images of mock-irradiated or irradiated cells immunostained for BrdU/ssDNA foci (red) are shown. Plot shows percentages of cells with more than 10 BrdU foci per nucleus after background subtraction. ( c ) Representative images of irradiated cells co-immunofluorescence stained with anti-cyclin A antibody (red) and anti-Rad51 antibody (green) are shown. Average numbers of Rad51 foci for cyclin A-positive (S/G2) nuclei are plotted after background subtraction. ( d – f ) Cells expressing rWT or 4D-EXO1 were pre-treated with CDK inhibitors (AZD5438 or roscovitine) or with DMSO as control, irradiated and assayed for RPA, BrdU or Rad51 foci, as indicated. Scale bar, 10 μm (for all images). All experiments were replicated three times. Error bars depict s.e.m. See also Supplementary Fig. 2 . Full size image Pharmacological inhibition of CDKs using AZD5438 or roscovitine severely impaired resection and HR ( Fig 2d–f ; Supplementary Fig. 2d–f ). Remarkably, 4D-EXO1 could partially override the effects of CDK inhibition. In accord with these results, expression of 4D-EXO1 could partially rescue decreased IR-induced RPA foci formation in CtIP- or DNA2-depleted cells ( Supplementary Fig. 2g,h ) demonstrating that phosphorylation of EXO1 is sufficient to trigger substantial resection in human cells, and therefore would be a step over which the cell must exercise stringent control as it traverses the cell cycle. Interaction of EXO1 and CDKs is obligatory for DNA end resection CDK–cyclin complexes, especially CDK2–cyclin A, bind to their substrates in a bipartite manner, with CDK binding to its phosphorylation site(s) and cyclin binding to distal RXL motif(s) called Cy [23] , [29] . We found that V5-EXO1 interacted with CDK1, CDK2, cyclin A and cyclin B in co-immunoprecipitation (co-IP) experiments ( Fig. 3a ), and these interactions were also seen by IP of endogenous EXO1 ( Supplementary Fig. 3a ). EXO1 bears two Cy motifs (at positions 204–206 and 293–295; Fig. 1d ). Mutation of both Cy motifs to Ala (CyMut) weakened interactions with CDK1 and particularly affected binding to CDK2 ( Fig. 3a ), as confirmed by reverse co-IP ( Supplementary Fig. 3b ). Importantly, mutation of both Cy motifs dramatically reduced EXO1 phosphorylation, as assessed by IP-westerns with both CDK substrate antibodies and the newly generated site-specific anti-p-T732 antibody ( Fig. 3b ). 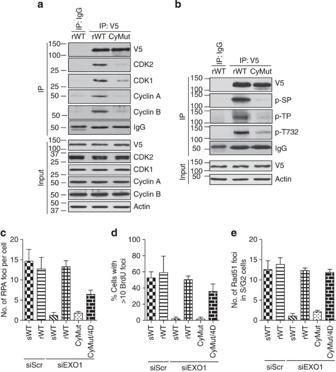Figure 3: Interaction of EXO1 and CDKs is obligatory for DNA end resection. (a) HEK-293 cells expressing V5-tagged wild-type EXO1 (rWT) or EXO1 with Cy (cyclin binding) sites mutated (CyMut) were synchronized in G2. Whole-cell extracts were immunoprecipitated (IP) with anti-V5 antibody and immunoprecipitates were probed by western blotting with the indicated antibodies. (b) HEK-293 cells expressing WT- or CyMut-EXO1 were synchronized in G2. EXO1 was immunoprecipitated (IP) with anti-V5 antibody and western blotted with anti-phospho-Ser (p-SP) or anti-phospho-Thr (p-TP) CDK substrate antibodies or with the site-specific anti-phospho-EXO1 (p-T732) antibody, as indicated. (c–e) U2OS cells were depleted of endogenous EXO1 using siRNA and complemented with siRNA-sensitive wild-type EXO1 (sWT) or siRNA-resistant wild-type EXO1 (rWT), Cy-mutant EXO1 (CyMut) or Cy-mutant EXO1 with phospho-mimic substitutions (CyMut/4D), as indicated. Cells were irradiated and assayed for RPA, BrdU/ssDNA or Rad51 foci, as indicated. All experiments were replicated three times. Error bars depict s.e.m. See alsoSupplementary Fig. 3. Cy mutations also resulted in severe defects in RPA, BrdU/ssDNA and Rad51 foci formation ( Fig 3c–e ; Supplementary Fig. 3c–f ). Strikingly, the resection and HR defects caused by Cy mutations could be rescued, at least partially, by phospho-mimic substitutions at the four C-terminal S/TP sites (CyMut/4D). Therefore, EXO1 interacts with CDK–cyclin complexes via its Cy motifs, and these interactions are required for EXO1 phosphorylation and DNA end resection; however, this requirement can be overridden by phospho-mimic substitutions on EXO1, unequivocally demonstrating that phosphorylation of EXO1 by CDKs is essential for resection in vivo . Figure 3: Interaction of EXO1 and CDKs is obligatory for DNA end resection. ( a ) HEK-293 cells expressing V5-tagged wild-type EXO1 (rWT) or EXO1 with Cy (cyclin binding) sites mutated (CyMut) were synchronized in G2. Whole-cell extracts were immunoprecipitated (IP) with anti-V5 antibody and immunoprecipitates were probed by western blotting with the indicated antibodies. ( b ) HEK-293 cells expressing WT- or CyMut-EXO1 were synchronized in G2. EXO1 was immunoprecipitated (IP) with anti-V5 antibody and western blotted with anti-phospho-Ser (p-SP) or anti-phospho-Thr (p-TP) CDK substrate antibodies or with the site-specific anti-phospho-EXO1 (p-T732) antibody, as indicated. ( c – e ) U2OS cells were depleted of endogenous EXO1 using siRNA and complemented with siRNA-sensitive wild-type EXO1 (sWT) or siRNA-resistant wild-type EXO1 (rWT), Cy-mutant EXO1 (CyMut) or Cy-mutant EXO1 with phospho-mimic substitutions (CyMut/4D), as indicated. Cells were irradiated and assayed for RPA, BrdU/ssDNA or Rad51 foci, as indicated. All experiments were replicated three times. Error bars depict s.e.m. See also Supplementary Fig. 3 . Full size image EXO1 phosphorylation promotes its recruitment to DSBs Next, we asked whether EXO1 phosphorylation might promote its recruitment to the sites of DSBs. We carried out live-cell imaging of green fluorescent protein (GFP)-tagged EXO1 at DNA breaks induced focally by laser micro-irradiation, as described before [20] . We have previously shown that EXO1 recruitment to breaks is significantly augmented in G2 relative to G1 (ref. 20 ). Therefore, to exclude any cell cycle effects, all GFP-EXO1 recruitment studies were carried out in cells synchronized in G2 ( Supplementary Fig. 4a ). The CDK inhibitor AZD5438 attenuated GFP-EXO1 accumulation indicating that CDK activity is important for damage-site localization of EXO1 ( Supplementary Fig. 4b ). In accord with this observation, the 4A-EXO1 mutant showed reduced accumulation at breaks while accumulation of 4D-EXO1 was augmented relative to WT-EXO1 ( Fig. 4a ). In parallel experiments, we quantified the recruitment of GFP-RPA to the sites of laser-induced DNA lesions in real time, as described previously [20] . We observed that GFP-RPA accumulation was attenuated in cells expressing 4A-EXO1 and augmented in cells expressing 4D-EXO1 ( Supplementary Fig. 4c ), indicating reduced and increased resection, respectively. Thus, phosphorylation of EXO1 by CDKs promotes its accumulation at DNA breaks that positively influences the extent of resection. 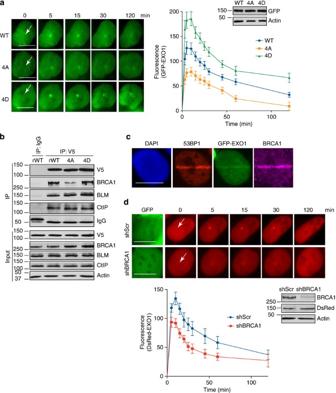Figure 4: EXO1 phosphorylation promotes its recruitment to DSBs. (a) U2OS cells expressing wild type (WT), phospho-mutant (4A) or phospho-mimic (4D) GFP-EXO1 were synchronized in G2 before laser micro-irradiation. Time-lapse images of accumulation of GFP-EXO1 (green) at DSBs induced by laser micro-irradiation (arrows) are shown. Plot shows recruitment of wild type or mutant forms of GFP-EXO1 after DNA damage. Western blot shows comparable levels of expression of GFP-EXO1. (b) HEK-293 cells expressing V5-tagged rWT-, 4A- or 4D-EXO1 were synchronized in G2. Whole-cell extracts were immunoprecipitated (IP) with anti-V5 antibody and immunoprecipitates were probed by western blotting with the indicated antibodies. (c) U2OS cells expressing GFP-EXO1 (green) were co-immunofluorescence stained with anti-53BP1 antibody (red) and anti-BRCA1 antibody (purple) 5 min after laser micro-irradiation. Nuclei were stained with 4',6-diamidino-2-phenylindole (blue). (d) U2OS cells with stable knockdown of BRCA1 (shBRCA1) or control cells (shScr), both expressing DsRed-EXO1, were synchronized in G2 before laser micro-irradiation. Cells transfected with shRNA vectors express GFP (green). Time-lapse images of accumulation of DsRed-EXO1 (red) at DSBs induced by laser micro-irradiation (arrows) are shown. Plot shows recruitment of DsRed-EXO1 after DNA damage. Western blot shows knockdown of BRCA1 and comparable levels of expression of DsRed-EXO1. Scale bar, 10 μm (for all images). All experiments were replicated three times. Error bars depict s.e.m. See alsoSupplementary Fig. 4. Figure 4: EXO1 phosphorylation promotes its recruitment to DSBs. ( a ) U2OS cells expressing wild type (WT), phospho-mutant (4A) or phospho-mimic (4D) GFP-EXO1 were synchronized in G2 before laser micro-irradiation. Time-lapse images of accumulation of GFP-EXO1 (green) at DSBs induced by laser micro-irradiation (arrows) are shown. Plot shows recruitment of wild type or mutant forms of GFP-EXO1 after DNA damage. Western blot shows comparable levels of expression of GFP-EXO1. ( b ) HEK-293 cells expressing V5-tagged rWT-, 4A- or 4D-EXO1 were synchronized in G2. Whole-cell extracts were immunoprecipitated (IP) with anti-V5 antibody and immunoprecipitates were probed by western blotting with the indicated antibodies. ( c ) U2OS cells expressing GFP-EXO1 (green) were co-immunofluorescence stained with anti-53BP1 antibody (red) and anti-BRCA1 antibody (purple) 5 min after laser micro-irradiation. Nuclei were stained with 4',6-diamidino-2-phenylindole (blue). ( d ) U2OS cells with stable knockdown of BRCA1 (shBRCA1) or control cells (shScr), both expressing DsRed-EXO1, were synchronized in G2 before laser micro-irradiation. Cells transfected with shRNA vectors express GFP (green). Time-lapse images of accumulation of DsRed-EXO1 (red) at DSBs induced by laser micro-irradiation (arrows) are shown. Plot shows recruitment of DsRed-EXO1 after DNA damage. Western blot shows knockdown of BRCA1 and comparable levels of expression of DsRed-EXO1. Scale bar, 10 μm (for all images). All experiments were replicated three times. Error bars depict s.e.m. See also Supplementary Fig. 4 . Full size image EXO1 is reported to interact with other proteins that control resection, namely, CtIP [30] and BLM [9] . We asked whether EXO1 phosphorylation might augment its recruitment to DSBs by facilitating some of these protein–protein interactions. We carried out co-IPs using extracts from HEK-293 cells synchronized in G2 and expressing WT-, 4A- or 4D-EXO1 ( Fig. 4b ). We observed interactions of EXO1 with CtIP and BLM but these interactions were not affected by the 4A mutations. Interestingly, we found that EXO1 also interacted with BRCA1, a key regulator of HR [31] , and this interaction was reduced by the 4A mutations ( Fig. 4b ), as confirmed by reverse co-IP ( Supplementary Fig. 4d ). Binding to BRCA1 was unaffected by irradiation of cells or by the presence of ethidium bromide ( Supplementary Fig. 4e ); thus, it is likely that these interactions are direct and not mediated by DNA. Notably, the BRCA1–EXO1 interaction was cell cycle dependent, showing a marked increase in cells synchronized in G2 ( Supplementary Fig. 4f ). BRCA1 binding was also seen on IP of endogenous EXO1 ( Supplementary Fig. 4g ). Co-IPs with single mutants of the four S/TP sites did not show greatly reduced BRCA1 binding, indicating that the interaction of EXO1 with BRCA1 involves more than one phospho-S/TP site ( Supplementary Fig. 4h ). In agreement with the observed interaction of EXO1 and BRCA1, we found that EXO1 rapidly co-localized with BRCA1 at sites of micro-laser-induced DNA lesions ( Fig. 4c ). BRCA1 has previously been shown to interact with phosphorylated CtIP and augment its localization at DNA breaks [12] , [13] , [32] , [33] . To see whether BRCA1 might have a similar role in EXO1 recruitment, we generated U2OS cells with stable short hairpin RNA (shRNA)-mediated BRCA1 knockdown and carried out live-cell imaging of DsRed-tagged EXO1 at DSBs induced by laser micro-irradiation, as described previously [20] ( Fig. 4d ). We found that EXO1 recruitment was reduced in BRCA1-depleted cells, indicating a partial dependency on BRCA1 for damage-site localization. We reasoned that if phospho-EXO1 was dependent on BRCA1 for recruitment to breaks, then 4D-EXO1 should not be able to complement the HR defect of BRCA1-deficient cells, although it is capable of alleviating HR defects caused by EXO1 depletion ( Fig. 2c ), mutation of Cy sites on EXO1 ( Fig. 3e ) or pharmacological inhibition of CDKs ( Fig. 2f ). Indeed, we found that expression of 4D-EXO1 could not correct defective Rad51 foci formation in BRCA1-depleted cells ( Supplementary Fig. 4i ) or reduce induction of radial chromosome structures [34] on irradiation ( Supplementary Fig. 4j ). In summary, although BRCA1 has a role in facilitating the recruitment of EXO1 to DSBs, whether the interactions between BRCA1 and EXO1 contribute to EXO1 recruitment remains to be determined. EXO1 phosphorylation regulates repair pathway choice Our results raised the possibility that phosphorylation of EXO1 by CDKs is a novel mechanism by which the cell exercises repair pathway choice. To address this, we used two different reporter assays to quantify the repair of I-SceI-induced DSBs by HR [17] or by NHEJ [35] . Cells bearing integrated HR or NHEJ reporters were depleted of endogenous EXO1 and complemented with siRNA-resistant WT-, 4A- or 4D-EXO1. Expression of 4A-EXO1 resulted in reduced levels of HR relative to WT-EXO1, while expression of 4D-EXO1 resulted in elevated levels of HR ( Fig. 5a ). Converse results were obtained with the NHEJ assay where expression of 4A-EXO1 resulted in increased levels of NHEJ relative to WT-EXO1 ( Fig. 5b ). The diametrically opposite effects of impaired EXO1 phosphorylation on HR and NHEJ clearly place this exonuclease at a pivotal point where the balance between these two repair pathways might be fine tuned by the cell. 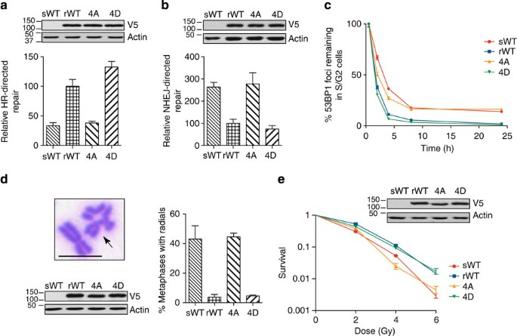Figure 5: EXO1 phosphorylation regulates repair pathway choice. (a) HR efficiency was measured by quantifying GFP expression (by flow cytometry) in MCF7 cells harbouring a DR-GFP reporter after transfection with an I-SceI plasmid. Cells were depleted of endogenous EXO1 using siRNA and complemented with sWT-, rWT-, 4A- or 4D-EXO1, as indicated. Plot shows HR-directed repair relative to rWT-EXO1-expressing cells. Western blot shows comparable levels of expression of siRNA-resistant EXO1. (b) NHEJ efficiency was measured by quantifying RFP expression in HEK-293 cells harbouring a GFP/RFP reporter after transfection with an I-SceI plasmid. The experiment was performed and data were plotted as ina. (c) U2OS cells depleted of endogenous EXO1 and expressing sWT-, rWT-, 4A- or 4D-EXO1 were irradiated and co-immunostained for 53BP1 foci and cyclin A (to demarcate cells in S/G2). Rates of DSB repair in S/G2 cells were determined by scoring 53BP1 foci in cyclin A-positive nuclei. Percent foci remaining was plotted against the indicated times post IR. (d) Percentages of metaphase spreads with one or more radial chromosomes (arrow) are plotted for irradiated U2OS cells with knockdown of endogenous EXO1 and with ectopic expression of wild type or mutant EXO1, as verified by western blotting. (e) Plot shows clonogenic survival of U2OS cells with knockdown of endogenous EXO1 and with ectopic expression of wild type or mutant EXO1, as verified by western blotting. Cells were synchronized in G2 and irradiated with the indicated doses before plating for colony formation. Scale bar, 5 μm. All experiments were replicated three times. Error bars depict s.e.m. See alsoSupplementary Fig. 5. Figure 5: EXO1 phosphorylation regulates repair pathway choice. ( a ) HR efficiency was measured by quantifying GFP expression (by flow cytometry) in MCF7 cells harbouring a DR-GFP reporter after transfection with an I-SceI plasmid. Cells were depleted of endogenous EXO1 using siRNA and complemented with sWT-, rWT-, 4A- or 4D-EXO1, as indicated. Plot shows HR-directed repair relative to rWT-EXO1-expressing cells. Western blot shows comparable levels of expression of siRNA-resistant EXO1. ( b ) NHEJ efficiency was measured by quantifying RFP expression in HEK-293 cells harbouring a GFP/RFP reporter after transfection with an I-SceI plasmid. The experiment was performed and data were plotted as in a . ( c ) U2OS cells depleted of endogenous EXO1 and expressing sWT-, rWT-, 4A- or 4D-EXO1 were irradiated and co-immunostained for 53BP1 foci and cyclin A (to demarcate cells in S/G2). Rates of DSB repair in S/G2 cells were determined by scoring 53BP1 foci in cyclin A-positive nuclei. Percent foci remaining was plotted against the indicated times post IR. ( d ) Percentages of metaphase spreads with one or more radial chromosomes (arrow) are plotted for irradiated U2OS cells with knockdown of endogenous EXO1 and with ectopic expression of wild type or mutant EXO1, as verified by western blotting. ( e ) Plot shows clonogenic survival of U2OS cells with knockdown of endogenous EXO1 and with ectopic expression of wild type or mutant EXO1, as verified by western blotting. Cells were synchronized in G2 and irradiated with the indicated doses before plating for colony formation. Scale bar, 5 μm. All experiments were replicated three times. Error bars depict s.e.m. See also Supplementary Fig. 5 . Full size image Next, we irradiated U2OS cells expressing WT-, 4A- or 4D-EXO1 and quantified the formation and dissolution of 53BP1 foci in G1 (cyclin A negative) versus S/G2 (cyclin A positive [28] ) nuclei to evaluate the effects of phospho-mutant versus phospho-mimic EXO1 on the overall kinetics of DSB repair ( Supplementary Fig. 5a ). Depletion of EXO1 had no discernible effect on G1 cells ( Supplementary Fig. 5b ) but resulted in a subtle but distinct DSB repair defect in S/G2 cells, as seen by comparing sWT with rWT ( Fig. 5c ). This defect could be corrected by expression of 4D-EXO1 but not by expression of 4A-EXO1. Consequently, irradiated cells expressing 4A-EXO1 exhibited a striking induction of radial chromosomes on IR ( Fig. 5d ), similar to that seen in BRCA1-deficient cells [34] ( Supplementary Fig. 4j ). Finally, cells expressing 4A-EXO1, but not those expressing 4D-EXO1, were sensitive to IR in the G2 phase of the cell cycle ( Fig. 5e ). It is important to point out that while attenuated repair and compromised survival in 4A-EXO1-expressing cells are clearly attributable to defective HR, the extent to which the altered balance between NHEJ and HR contributes to these defects remains to be elucidated. Taken together, these results demonstrate that EXO1 phosphorylation is critical for DSB repair in S and G2 phases, maintenance of genomic integrity and long-term cell survival in response to DNA damage. It is well established that CDKs regulate repair pathway choice by controlling the first step in resection (initiation) by phosphorylating CtIP at seven S/TP sites [10] , [11] , [12] , [13] , [14] , [15] and NBS1 at a single site [16] . The second step in resection (long-range resection) is indispensable for successful HR [3] , [4] . Currently, it is not known whether CDKs regulate this key step in human cells. Our results uncover a novel mechanism by which CDKs regulate the second step in resection by modifying EXO1, an exonuclease with critical functions in long-range resection. EXO1 belongs to the RAD2/XPG family of nucleases and displays 5′–3′ exonuclease activity on single- and double-stranded DNA substrates, as well as flap structure-specific endonuclease activity. EXO1 plays important roles in DNA mismatch repair (MMR), mitotic and meiotic recombination, replication and telomere homoeostasis [36] . EXO1 is phosphorylated at S714 by ataxia-telangiectasia mutated (ATM) in response to DSBs [17] and by ataxia-telangiectasia- and Rad3-related (ATR) in response to replication stress [26] , which influences its activity and stability, respectively. The amino-terminal 300 amino acids of EXO1 encompassing its nuclease domain are highly conserved across species and share common sequences with other RAD2 nucleases [24] . In contrast, the carboxy-terminal region of EXO1 is divergent and mediates interactions with the 14-3-3 checkpoint regulatory proteins [37] , the proliferating cell nuclear antigen [38] and MMR proteins such as MutSα [36] . In the context of MMR, it has been proposed that the C terminus forms an unstructured regulatory domain that interacts with the N-terminal catalytic domain resulting in autoinhibition of EXO1; interaction of the C terminus with MutSα not only couples EXO1 to the MMR machinery but also relieves inhibition of the catalytic domain [24] . How EXO1 is regulated in the context of HR and whether its C terminus plays any role in such regulation is currently not well understood. We find that the C-terminal domain of EXO1 is phosphorylated by CDKs 1 and 2 at S639, T732, S815 and T824 during S and G2 phases of the cell cycle. Phosphorylation of these four sites promotes DNA end resection and DSB repair by HR, thereby preserving chromosomal integrity and promoting survival on DNA damage. Further bolstering the connection between CDKs and EXO1, we find that Cy-mutant EXO1 (defective in cyclin-CDK binding) phenocopies 4A-EXO1 (all four phosphorylation sites mutated) in terms of resection and HR defects. Our results indicate that phosphorylation of EXO1 promotes end resection, in part, by augmenting the localization of EXO1 to DNA breaks possibly via interactions with BRCA1. The BRCA1–EXO1 interaction is limited to S/G2 phases, and this might serve to restrict resection to the post-replicative phases of the cell cycle. As even individual mutations of these four phosphorylation sites result in pronounced resection defects, it is possible that, individually, these four sites have additional and non-redundant functions that are yet to be discovered. Such a situation exists in the regulation of CtIP by CDKs. CtIP is phosphorylated at multiple sites by CDKs, which promote resection in distinct ways such as facilitating interactions with Nbs1 and phosphorylation by ATM (ref. 14 ), promoting phosphorylation by ATR (refs 5 , 11 , 39 ) and augmenting damage-site localization via interaction with BRCA1 (refs 12 , 13 , 15 , 40 ). A key question for the future is to determine the extent to which this type of regulation applies to EXO1. With regard to the recruitment of EXO1 to DNA breaks, BRCA1 could also promote this step indirectly by augmenting CtIP binding [40] or antagonizing 53BP1-RIF1 binding [41] to DNA ends. It is important to point out that combined mutation of all four CDK phosphorylation sites or depletion of BRCA1 attenuates, but does not abolish, damage-site localization of EXO1. Therefore, it is likely that BRCA1 binding is only one mechanism by which EXO1 is recruited to DNA breaks and other mechanism(s), perhaps involving interactions with other resection proteins, are yet to be elucidated. In this regard, yeast MRX and Sae2 have been reported to promote the binding of Exo1 to DNA ends in vitro [42] . We too find that EXO1 binds to CtIP and BLM in vivo , as reported by others [9] , [30] , although binding is not affected by the phospho-site mutations. Thus, it is plausible that additional protein–protein interactions could serve to stabilize EXO1 at DNA breaks independently of these four phospho-S/TP sites. It is interesting that single mutants of EXO1, unlike 4A-EXO1, show no or minimal loss of BRCA1 binding, yet exhibit pronounced resection defects. Although we cannot rule out subtle but critical BRCA1 interaction defects of the single EXO1 mutants that would not be revealed by co-IPs, this observation supports the hypothesis that additional, non-redundant mechanisms contribute to the resection defects of individual EXO1 mutants. Elucidating additional functions for the identified phosphorylation sites on EXO1 is an important task for the future, and our study sets the stage for investigating such mechanisms. Finally, our results demonstrating regulation of long-range resection by CDKs in human cells have some precedence in yeast where Cdk1-dependent Dna2 phosphorylation has been shown to regulate DNA end resection [43] . In summary, our findings indicate that phosphorylation of EXO1 by CDKs in S/G2 phases stimulates resection, in part, by promoting EXO1 accumulation at DSBs, and regulation of long-range resection in this manner is critical for repair pathway choice, maintenance of genomic integrity and long-term survival in the face of genomic insults. Cell culture and CDK inhibitor treatments U2OS and HEK-293 cells (obtained from the American Type Culture Collection) were maintained in α-MEM and DMEM medium, respectively, supplemented with 10% fetal bovine serum and penicillin/streptomycin in a humidified atmosphere with 5% CO 2 . A U2OS line with stable shRNA-mediated knockdown of BRCA1 was generated by transfection with a pGIPZ vector (5′-TATGTGGTCACACTTTGTG-3′; No. : V2LHS_254648, Thermo Scientific) using Lipofectamine2000 (Invitrogen) followed by selection and continued maintenance in puromycin (1 μg ml −1 , Invitrogen). Control cells were generated by transfection with a pGIPZ vector expressing scrambled shRNA (No. : RHS4346, Thermo Scientific). For CDK inhibition, cells were incubated with 2 μM AZD5438 (Selleck) or 10 μM roscovitine (Sigma) for 5 h before cells were harvested or irradiated. Cell cycle synchronization and flow cytometry HEK-293 cells were synchronized in G1 by treatment with aphidicolin (2 μg ml −1 , Sigma) for 16 h and then released into regular media for either 5 h (S phase) or 10 h (G2 phase) [19] . Alternatively, HEK-293 cells were synchronized in late G2 by treatment with nocodazole (100 ng ml −1 , Sigma) for 16 h. Cell cycle stage was determined by flow cytometry using a BD CYTOMICS FC500 Flow Cytometer (Becton, Dickinson and Company). Cloning and mutagenesis EXO1b was subcloned from Flag2-EXO1 (ref. 17 ) into pDONR221 (Invitrogen) using the Gateway BP Clonase II enzyme mix (Invitrogen). Site-directed mutagenesis of EXO1 was carried out using the QuikChange II XL Site-Directed Mutagenesis kit (Stratagene); see Supplementary Table 1 for primer sequences. EXO1 was then transferred to pLenti6.3/V5-DEST (Invitrogen) for C-terminal V5-tagged fusion protein expression. Transfection of cells Depletion of EXO1 or CDKs was carried out by transfection with appropriate siRNAs ( Supplementary Table 2 ; Invitrogen) using electroporation (Amaxa) for U2OS cells and Lipofectamine2000 (Invitrogen) for HEK-293 cells; cells were harvested 48 h later to verify knockdown by western blotting. Cells were transfected with scrambled siRNA as controls. For expression of tagged proteins, cells were transfected with the appropriate expression plasmid and harvested after 24–48 h. For ectopic expression of EXO1 in cells with knockdown of endogenous EXO1 or CDKs, cells were transfected with the expression plasmid 24 h after siRNA transfection. Western blotting and antibodies Nuclear extracts for western blotting were prepared by re-suspending cell pellets in hypotonic lysis buffer (10 mM Tris–HCl pH 7.5, 1.5 mM MgCl 2 , 5 mM KCl, protease and phosphatase inhibitors), followed by nuclear extraction buffer (50 mM Tris–HCl pH 7.5, 0.5 M NaCl, 2 mM EDTA, 10% sucrose, 10% glycerol, protease and phosphatase inhibitors) [19] . The following primary antibodies were used: V5 (Invitrogen), Phospho-(Thr) CDK substrate, phospho-(Ser) CDK substrate, CHK1, phospho-CHK1 (S317), phospho-CHK2 (T68) (Cell Signaling), CDK1 (C-19), CDK2 (H-298, D-12), Rad51 (H-92), cyclin B1 (H-433), 53BP1 (H-300; Santa Cruz), actin (Sigma), RPA (Calbiochem), BrdU (Becton, Dickinson and Company), cyclin A (6E6), GFP (Abcam), BRCA1, EXO1 monoclonal (ThermoFisher), EXO1 polyclonal, CtIP, BLM, CHK2 (Bethyl), DsRed (Clontech) and Ku80 (a kind gift from Dr BP Chen). The following secondary antibodies were used: horseradish peroxidase-conjugated secondary antibodies (Bio-Rad) and Alexa488/568/647-conjugated secondary antibodies (Invitrogen). Antibody dilutions and catalogue numbers are provided in Supplementary Table 3 . Rabbit polyclonal phospho-specific antibody against p-T732 of EXO1 was generated by Abmart using the phospho-peptide NH 2 -Cys-FSKKD(pT)PLRNK-COOH, where pT indicates phospho-Thr. Uncropped scans of western blots are shown in Supplementary Fig. 6 . Immunoprecipitation Whole-cell extracts were prepared in lysis buffer (20 mM Tris–HCl pH 7.5, 80 mM NaCl, 2 mM EDTA, 10% glycerol, 0.2% NP-40) with additional protease and phosphatase inhibitors. Antibodies were bound to Dynabeads (Invitrogen) and beads were incubated overnight with cell extracts, following the manufacturer’s protocol. Beads were washed extensively in lysis buffer and then boiled in 1 × SDS loading buffer before western blotting. Normal mouse IgG (Santa Cruz) was used for control immunoprecipitations. Irradiation of cells Cells were irradiated with gamma rays from a caesium source (JL Shepherd and Associates). For laser irradiation, cells were pre-sensitized by overnight incubation with BrdU (10 μg ml −1 ) and then micro-irradiated with a pulsed nitrogen laser (Spectra-Physics; 365 nm, 10 Hz) with output set at 70% of the maximum [20] . Cells were maintained at 37 °C in 35 mm glass-bottom culture dishes (MatTek Cultureware) during micro-irradiation and image acquisition; the growth medium was replaced by CO 2 -independent medium (Invitrogen) before irradiation. Immunofluorescence staining Cells were seeded onto glass chamber slides (Lab-Tek) and immunostained with anti-RPA antibody or co-immunostained with anti-Rad51 and anti-cyclin A antibodies 3 h after irradiation with 6 Gy. Cells were fixed with 4% paraformaldehyde/PBS and permeabilized with 0.5% Triton X-100 before incubation with antibodies [19] . To obtain clear RPA foci, cells were subject to in situ fractionation [44] . The average number of RPA foci per nucleus or mean Rad51 foci for cyclin A-positive (S/G2) nuclei [28] was determined after scoring at least 50 nuclei and subtracting background (average numbers of foci in mock-irradiated cells). For quantifying DSB repair kinetics, cells were co-immunostained with anti-53BP1 and anti-cyclin A antibodies at different time points post irradiation (1 Gy), as described previously [35] . The average numbers of 53BP1 foci for cyclin A-positive (S/G2) and cyclin A-negative (G1) nuclei were determined after scoring at least 50 nuclei and subtracting background. Images were captured using a Leica DH5500B fluorescence microscope (× 40 objective lens) coupled to a Leica DFC340 FX camera using Leica Application Suite v3 acquisition software. BrdU/ssDNA assay Cells grown in the presence of 10 μM BrdU (Sigma) for 16 h were irradiated with 10 Gy of gamma rays and fixed 1 h after irradiation. Cells were immunofluorescence stained with anti-BrdU antibody under non-denaturing conditions (to detect BrdU incorporated into ssDNA) [20] . For clarifying BrdU/ssDNA foci, cells were subject to in situ fractionation [44] . The percentage of BrdU-positive cells (cells with 10 or more foci) was determined after scoring at least 50 nuclei and subtracting background. HR and NHEJ assays To measure HR, GFP expression in MCF7 cells with an integrated DR-GFP reporter was quantified by flow cytometry [17] . To measure NHEJ, red fluorescent protein (RFP) expression in HEK-293 cells with an integrated GFP-to-RFP reporter was quantified by flow cytometry. For both assays, cells were co-transfected with siRNA against endogenous EXO1 and the V5-EXO1 expression plasmid; after 24 h, cells were transfected with an I-SceI plasmid, and GFP or RFP expression was quantified by flow cytometry after an additional 72 h. GFP+ or RFP+ frequencies were corrected for transfection efficiencies (measured simultaneously by parallel transfection with a wild-type GFP expression vector). Metaphase chromosome preparations Cells were irradiated with 6 Gy of gamma rays. Colcemid (Sigma), along with 1 mM caffeine (Sigma) to bypass G2/M arrest, was added at 8 h post IR. Metaphase chromosome spreads were prepared after 16 h and scored for triradial and quadriradial chromosomes [45] . Live-cell imaging combined with laser micro-irradiation Cells were transfected with GFP-EXO1, GFP-RPA or DsRed-EXO1 constructs, laser micro-irradiated and time-lapse imaged, and the fluorescence intensities of micro-irradiated areas were plotted after background subtraction (fluorescence intensities of unirradiated areas) [20] , [46] . In brief, cells were irradiated and live-cell images were taken using a pulsed nitrogen laser (Spectra-Physics; 365 nm, 10 Hz) coupled to a Carl Zeiss Axiovert 200 M microscope (× 63 oil immersion objective). Fluorescence intensities were determined using Axiovision software v4.8 that converts signal intensities of accumulated GFP or DsRed into numerical values (arbitrary units). The fluorescence intensity of an unirradiated region was subtracted from the fluorescence intensity of the micro-irradiated area for each nucleus at each time point to compensate for nonspecific fluorescence bleaching during repeated image acquisition. Mean value of the fluorescence intensities for each time point was calculated from at least 40 independent measurements. Total increase in fluorescence signal (after background subtraction) was plotted versus time. Colony formation assays Cells were synchronized in G2 and irradiated with the indicated doses of gamma rays. After 4 h, cells were plated in triplicate onto 60 mm dishes (1,000 cells per dish). Surviving colonies were stained with crystal violet ~10–14 days later. How to cite this article: Tomimatsu, N. et al . Phosphorylation of EXO1 by CDKs 1 and 2 regulates DNA end resection and repair pathway choice. Nat. Commun. 5:3561 doi: 10.1038/ncomms4561 (2014).